Recovery from chronic monocular deprivation following reactivation of thalamocortical plasticity by dark exposure Chronic monocular deprivation induces severe amblyopia that is resistant to spontaneous reversal. However, dark exposure initiated in adulthood reactivates synaptic plasticity in the visual cortex and promotes recovery from chronic monocular deprivation in Long Evans rats. Here we show that chronic monocular deprivation induces a significant decrease in the density of dendritic spines on principal neurons throughout the deprived visual cortex. Nevertheless, dark exposure followed by reverse deprivation promotes the recovery of dendritic spine density of neurons in all laminae. Importantly, the ocular dominance of neurons in thalamo-recipient laminae of the cortex, and the amplitude of the thalamocortical visually evoked potential recover following dark exposure and reverse deprivation. Thus, dark exposure reactivates widespread synaptic plasticity in the adult visual cortex, including thalamocortical synapses, during the recovery from chronic monocular deprivation. The ocular dominance of binocular neurons in the primary visual cortex is maintained postnatally by a competition between synapses serving the two eyes. Brief monocular deprivation in juveniles induces a shift in ocular dominance, mediated by a rapid decrease in the strength of excitatory synapses serving the deprived eye [1] . Deprived eye depression shares many characteristics with the homosynaptic long-term depression (LTD) of excitatory synapses that is induced by low-frequency stimulation [2] , [3] , [4] , including a decline over the course of postnatal development [5] , [6] . Both deprived eye depression and LTD are induced by decorrelation of pre- and postsynaptic activity [3] , [7] , and the expression is mediated by endocytosis of the AMPA (α-amino-3-hydroxy-5-methyl-4-isoxazolepropionic acid) subtype of glutamate receptor [4] . Importantly, the deprived eye depression induced by monocular deprivation occludes subsequent LTD of excitatory synaptic transmission in slices of rat visual cortex [2] . Extending the duration of monocular deprivation in juvenile mice reveals a delayed potentiation of the response to stimulation of the non-deprived eye [1] , [8] . The majority of excitatory synaptic transmission in the mammalian cortex occurs on the heads of dendritic spines. In the visual cortex, ∼ 95% of all dendritic spines form synapses, and spine head volume is positively correlated with the area of the postsynaptic density [9] . Manipulations that regulate synaptic strength, such as sensory input and changes in arousal state, induce changes in dendritic spine morphology and spine density [10] , [11] , [12] . Indeed, LTD in hippocampal slice cultures is accompanied by a retraction in dendritic spines [13] and a decrease in the number of contacts between presynaptic boutons and postsynaptic spines [14] , [15] . In addition, low-frequency stimulation of excitatory synapses in the rat hippocampus activates the NMDA ( N -Methyl- D -aspartic acid or N -Methyl- D -aspartate) subtype of glutamate receptor, and subsequent reduction in spine heads [16] and depolymerization of actin [17] , [18] . Robust anatomical changes are also induced in the juvenile visual cortex by monocular deprivation. For example, in juvenile mice, monocular deprivation induces an initial decrease in the density of dendritic spines on the apical dendrites of supragranular neurons, which recovers following prolongation of the monocular deprivation [19] . Monocular deprivation also increases the turnover on dendritic spines in layers II/III and V on layer V apical dendrites in juvenile mice [20] . In contrast, experience-dependent anatomical plasticity is extremely limited in adult rodent visual cortex [19] , [20] , [21] , but can be encouraged with repeated episodes of monocular deprivation [22] or enzymatic degradation of the extracellular matrix [23] . The developmental constraint on cortical plasticity may limit the ability to recover from monocular deprivation. For example, the ocular dominance shift induced by brief monocular deprivation in juvenile kittens and ferrets is rapidly reversed if the occlusion is removed early in postnatal development [24] , [25] , [26] . In contrast, chronic monocular deprivation in rats, from eye opening to adulthood, induces a significant shift in ocular dominance that does not reverse spontaneously following removal of the occlusion [23] , [27] , [28] . Chronic monocular deprivation would be expected to induce considerable depression and subsequent elimination of deprived eye synapses, imposing additional obstacles to recovery. Indeed, a significant decrease in thalamocortical afferents serving the deprived eye is observed following prolonged monocular deprivation in monkeys, cats and mice, due to a retraction of preexisting afferents or an inhibition of axonal outgrowth [29] , [30] , [31] , [32] , [33] . However, we have recently reported that robust ocular dominance plasticity can be reactivated in adult Long Evans rats by binocular visual deprivation through dark exposure. Dark exposure in adulthood promotes the recovery of visual functions following chronic monocular deprivation [27] . This complements a growing list of experimental interventions shown to reactivate synaptic plasticity in the adult visual cortex [23] , [28] , [34] . The ability to recover from severe deprivation amblyopia suggests that some feedforward excitation persists following chronic monocular deprivation; however, this prediction is at odds with the expectation that chronic monocular deprivation would significantly degrade anatomical connectivity in the pathway serving the chronically deprived eye. Therefore, we used an unbiased labelling method (DiOlistic staining [35] ) to track the density and morphology of dendritic spines along the basolateral dendrites of pyramidal neurons, which receive substantial feedforward excitation [36] . Following chronic monocular deprivation, from eye opening to adulthood, we observed a significant, parallel decrease in dendritic spine density throughout the depth of the visual cortex. Nevertheless, presentation of visual stimuli to the chronically deprived eye continued to evoke neuronal spiking and thalamocortical synaptic potentials. Dark exposure followed by reverse deprivation promoted the recovery of dendritic spine densities throughout the depth of the visual cortex, and the recovery of visually evoked activity including thalamocortical synaptic potentials. We conclude that dark exposure in adulthood reactivates widespread anatomical and physiological plasticity in the visual cortex, including thalamocortical synapses, to promote the recovery from chronic monocular deprivation. Dendritic spine density increases during amblyopia recovery We used visually evoked potentials (VEPs) acquired from layer IV of the binocular visual cortex in response to high-contrast horizontal gratings (0.02–0.04 cycles/degree, 96% contrast, reversing at 1 Hz) to track the physiological response to manipulations of visual input in Long Evans rats ( Fig. 1 ). The contralateral bias of the rodent visual system results in a twofold larger VEP amplitude in response to stimulation of the contralateral eye relative to the ipsilateral eye. Chronic monocular deprivation of the dominant contralateral eye, from eye opening to adulthood (postnatal day P14 to postnatal day 148±11.65), induced a significant decrease in the VEP contralateral bias. Binocular visual deprivation, through dark exposure, followed by reverse deprivation in adulthood (open the chronically deprived eye and close the chronically non-deprived eye), reversed the decrease in the VEP contralateral bias (VEP amplitude in response to stimulation of contralateral/ipsilateral eye, average±s.e.m. : control=2.16±0.16; chronic monocular deprivation (cMD)=0.37±0.06; chronic monocular deprivation+dark exposure+reverse deprivation (cMD DE-RD)=1.93±0.05; one-way analysis of variance (ANOVA), F( 2,14 )=94.5117, P <0.0001, n =5 each group; Fig. 1c ). The reversible regulation of the VEP contralateral bias was reflected in the VEP evoked by stimulation of the deprived eye (contralateral eye normalized to amplitude of contralateral+ipsilateral, average±s.e.m. : control=0.68±0.02; cMD=0.27±0.03; cMD DE-RD=0.66±0.01; one-way ANOVA, F( 2,14 )=155.2638, P <0.0001; Fig. 1d ) and non-deprived (ipsilateral) eye (control=0.32±0.02; cMD=0.73±0.03; cMD DE-RD=0.34±0.01; one-way ANOVA, F( 2,14 )=114.2875, P <0.0001; Fig. 1e ). 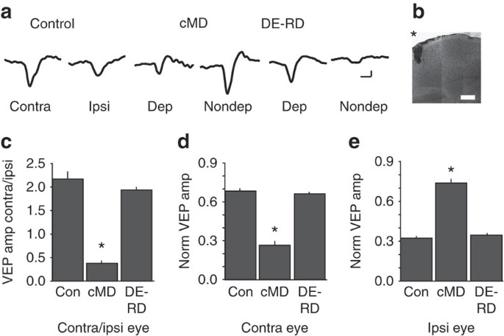Figure 1: Reversible regulation of VEP contralateral bias in adults. (a) Representative layer IV VEP waveforms evoked by visual stimulation of the contralateral (contra) and ipsilateral (ipsi) eye in adults with binocular vision (control) chronic monocular deprivation (cMD), cMD followed by dark exposure and reverse deprivation (DE-RD; average of 100 presentations of 0.02–0.04 cycles/degree horizontal gratings, 96% contrast, reversing at 1 Hz). Scale bars, 50 ms, 50 μV. (b) Photomontage of nissl stain confirms placement of recording electrode (*) in layer IV of visual cortex. Scale bar, 500 μm. (c) Chronic monocular deprivation induces a significant reduction in VEP contralateral bias (VEP amplitude (amp) in response to stimulation of contralateral eye/ipsilateral eye), which recovers following dark exposure and reverse deprivation (average±s.e.m.; one-way ANOVA, F(2,14)=94.5117,P<0.0001,n=5 each group). (d) Reversible regulation of the deprived eye VEP amplitude (one-way ANOVA, F(2,14)=155.2638,P<0.0001). (e) Reversible regulation of the non-deprived eye VEP amplitude (one-way ANOVA, F(2,14)=114.2875,P<0.0001); *P<0.05 versus control, Tukey–Kramer honestly significant differencepost hoc). Figure 1: Reversible regulation of VEP contralateral bias in adults. ( a ) Representative layer IV VEP waveforms evoked by visual stimulation of the contralateral (contra) and ipsilateral (ipsi) eye in adults with binocular vision (control) chronic monocular deprivation (cMD), cMD followed by dark exposure and reverse deprivation (DE-RD; average of 100 presentations of 0.02–0.04 cycles/degree horizontal gratings, 96% contrast, reversing at 1 Hz). Scale bars, 50 ms, 50 μV. ( b ) Photomontage of nissl stain confirms placement of recording electrode (*) in layer IV of visual cortex. Scale bar, 500 μm. ( c ) Chronic monocular deprivation induces a significant reduction in VEP contralateral bias (VEP amplitude (amp) in response to stimulation of contralateral eye/ipsilateral eye), which recovers following dark exposure and reverse deprivation (average±s.e.m. ; one-way ANOVA, F( 2,14 )=94.5117, P <0.0001, n =5 each group). ( d ) Reversible regulation of the deprived eye VEP amplitude (one-way ANOVA, F( 2,14 )=155.2638, P <0.0001). ( e ) Reversible regulation of the non-deprived eye VEP amplitude (one-way ANOVA, F( 2,14 )=114.2875, P <0.0001); * P <0.05 versus control, Tukey–Kramer honestly significant difference post hoc ). Full size image To identify changes in the anatomy of excitatory circuitry that may underlie the recovery from chronic monocular deprivation, we tracked the density and morphology of dendritic spines in the adult visual cortex ( Fig. 2 ). We focused on basolateral dendrites of principal neurons, which receive significant feedforward excitatory input [36] and limited our analysis to dendrites that could be traced back to pyramidal neuron cell bodies in the binocular primary visual cortex. Dendritic spines were binned in 25 micron segments, starting at the cell body, and analysed across ∼ 100 microns of the basolateral dendrite. Chronic deprivation of the contralateral eye significantly decreased the density of dendritic spines in the deprived visual cortex. Surprisingly, dendritic spine densities were unchanged following dark exposure; however, dark exposure followed by reverse deprivation in adulthood promoted an increase in dendritic spine densities (average spines/micron across 25 micron segments±s.e.m. : 0–25 μm control=0.16±0.02 (19,8); chronic MD=0.09±0.01 (24,9); cMD DE=0.08±0.01 (20,8); cMD DE-RD=0.13±0.02 (16,6); n =neurons, subjects; 25–50 μm control=0.65±0.04; chronic MD=0.36±0.05; cMD DE=0.36±0.05; cMD DE-RD=0.59±0.07; 50–75 μm control=0.90±0.05; chronic MD=0.52±0.05; cMD DE=0.52±0.05; cMD DE-RD=0.73±0.08; 75–100 μm: control=1.01±0.04; chronic MD=0.63±0.07; cMD DE=0.59±0.08; cMD DE-RD=0.76±0.07; Fig. 2c ). 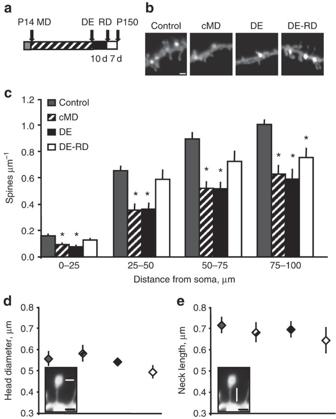Figure 2: Reversible regulation of dendritic spine density in adult visual cortex. (a) Experimental timeline. Chronic monocular deprivation (cMD) from postnatal day 14–150 (P14–P150) was followed by 10 days of dark exposure (DE) and 7 days of reverse deprivation (RD). (b) Representative DiI-labelled basolateral dendrites of pyramidal neurons in deprived binocular visual cortex from adult with binocular vision (Control), chronic monocular deprivation (cMD), chronic monocular deprivation plus dark exposure (DE) and chronic monocular deprivation plus dark exposure and reverse deprivation (DE-RD). The dendritic segment shown is 75–100 μm from the cell body. Scale bar, 2.5 μm. (c) Chronic monocular deprivation induces a significant reduction in spine density in all dendritic segments, which is unchanged following dark exposure. Dark exposure followed by reverse deprivation increased dendritic spine densities in proximal (0–75 μm) segments (average spines/micron across 25 micron segments±s.e.m.; one-way ANOVAs: 0–25 μm F(3,78)=5.7840,P=0.0013; 25–50 μm F(3,78)=7.1713,P<0.0001; 50–75 μm F(3,75)=10.0410,P<0.0001; 75–100 μm F(3,63)=8.2569,P=0.0001; *P<0.05 versus within-segment control, Tukey–Kramer honestly significant differencepost hoc);n(neurons, subjects): Con (19,8), cMD (24,9), DE (20,8), DE-RD(16,6)). (d) No significant difference in dendritic spine-head diameters across experimental conditions. (e) No significant difference in dendritic spine lengths across experimental conditions. Insets: White lines depict area used for measurements of spine-head diameter and neck length. Scale bar, 1 μm. Figure 2: Reversible regulation of dendritic spine density in adult visual cortex. ( a ) Experimental timeline. Chronic monocular deprivation (cMD) from postnatal day 14–150 (P14–P150) was followed by 10 days of dark exposure (DE) and 7 days of reverse deprivation (RD). ( b ) Representative DiI-labelled basolateral dendrites of pyramidal neurons in deprived binocular visual cortex from adult with binocular vision (Control), chronic monocular deprivation (cMD), chronic monocular deprivation plus dark exposure (DE) and chronic monocular deprivation plus dark exposure and reverse deprivation (DE-RD). The dendritic segment shown is 75–100 μm from the cell body. Scale bar, 2.5 μm. ( c ) Chronic monocular deprivation induces a significant reduction in spine density in all dendritic segments, which is unchanged following dark exposure. Dark exposure followed by reverse deprivation increased dendritic spine densities in proximal (0–75 μm) segments (average spines/micron across 25 micron segments±s.e.m. ; one-way ANOVAs: 0–25 μm F( 3,78 )=5.7840, P =0.0013; 25–50 μm F( 3,78 )=7.1713, P <0.0001; 50–75 μm F( 3,75 )=10.0410, P <0.0001; 75–100 μm F( 3,63 )=8.2569, P =0.0001; * P <0.05 versus within-segment control, Tukey–Kramer honestly significant difference post hoc ); n (neurons, subjects): Con (19,8), cMD (24,9), DE (20,8), DE-RD(16,6)). ( d ) No significant difference in dendritic spine-head diameters across experimental conditions. ( e ) No significant difference in dendritic spine lengths across experimental conditions. Insets: White lines depict area used for measurements of spine-head diameter and neck length. Scale bar, 1 μm. Full size image Approximately 50% of dendritic spines on principal neurons of the deprived visual cortex persisted following chronic monocular deprivation. To test whether the morphology of the spared dendritic spines revealed evidence of neuronal compensation for the spine loss, we measured the head diameter and neck length of residual spines across all experimental conditions. No change in the average diameter of spine heads was observed following chronic monocular deprivation, dark exposure or dark exposure followed by reverse deprivation (average spine head diameter±s.e.m. : control=0.56±0.03 (19,8); chronic MD=0.59±0.03 (24,9); cMD DE=0.54±0.01 (20,8); cMD DE-RD=0.50±0.03 (16,6); n =neurons, subjects; Fig. 2d ). Similarly, no change in dendritic spine neck lengths was observed across experimental conditions (average spine neck length±s.e.m. : control=0.72±0.03; chronic MD=0.69±0.04; cMD DE=0.70±0.03; cMD DE-RD=0.65±0.05; Fig. 2e ). Complementary changes in dendritic spine density were not observed in the non-deprived visual cortex (ipsilateral to the occluded eye), suggesting that deprivation of the ipsilateral input was insufficient to trigger elimination of excitatory synapses ( Fig. 3 ). Nevertheless, dark exposure and reverse deprivation induced a significant decrease in dendritic spine density in the non-deprived visual cortex, suggesting that the reactivation of synaptic plasticity by dark exposure promotes synapse elimination following deprivation of the dominant input (average spines/micron across 25 micron segments±s.e.m. : 0–25 μm control=0.16±0.02 (16,7); Nondep=0.16±0.02 (19,8); Nondep DE=0.13±0.01 (26,8); Nondep DE-RD=0.08±0.02 (9,4); 25–50 μm control=0.67±0.04, Nondep=0.64±0.06, Nondep DE=0.52±0.04, Nondep DE-RD=0.44±0.08; 50–75 μm control=0.93±0.06, Nondep=0.82±0.04, Nondep DE=0.74±0.05, Nondep DE-RD=0.54±0.09 spines μm −1 ; 75–100 μm: control=1.04±0.03, Nondep=0.92±0.04, Nondep DE=0.86±0.05, Nondep DE-RD=0.57±0.09 spines μm −1 ; n =neurons, subjects). 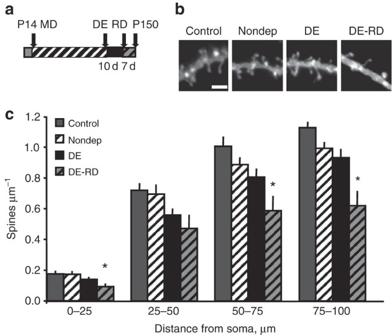Figure 3: Relative stability of dendritic spine density in the non-deprived adult visual cortex. (a) Experimental timeline. (b) Representative DiI-labelled basolateral dendrites of pyramidal neurons in non-deprived binocular visual cortex from adult with binocular vision (Control), chronic monocular deprivation (Nondep), chronic monocular deprivation plus dark exposure (DE) and chronic monocular deprivation plus dark exposure and reverse deprivation (DE-RD). In each case, the dendritic segment shown is 75–100 μm from the cell body. Scale bar, 2.5 μm. (c) No significant differences in spine density in any dendritic segments following chronic monocular deprivation or dark exposure. Dark exposure and reverse deprivation induce a reduction in dendritic spine density in all dendritic segments (average spines/micron across 25 micron segments±s.e.m.; one-way ANOVAs: 0–25 μm F(3,69)=3.4272,P=0.0220; 25–50 μm F(3,69)=3.5132,P=0.0199; 50–75 μm F(3,68)=5.6344,P=0.0017; 75–100 μm: F(3,61)=9.7476,P<0.0001, *P<0.05 versus control, Tukey–Kramer honestly significant differencepost hoc;n(neurons, subjects): Control (19,8), Nondep (24,9), DE (20,8), DE-RD (16,6). Figure 3: Relative stability of dendritic spine density in the non-deprived adult visual cortex. ( a ) Experimental timeline. ( b ) Representative DiI-labelled basolateral dendrites of pyramidal neurons in non-deprived binocular visual cortex from adult with binocular vision (Control), chronic monocular deprivation (Nondep), chronic monocular deprivation plus dark exposure (DE) and chronic monocular deprivation plus dark exposure and reverse deprivation (DE-RD). In each case, the dendritic segment shown is 75–100 μm from the cell body. Scale bar, 2.5 μm. ( c ) No significant differences in spine density in any dendritic segments following chronic monocular deprivation or dark exposure. Dark exposure and reverse deprivation induce a reduction in dendritic spine density in all dendritic segments (average spines/micron across 25 micron segments±s.e.m. ; one-way ANOVAs: 0–25 μm F (3,69) =3.4272, P =0.0220; 25–50 μm F (3,69) =3.5132, P =0.0199; 50–75 μm F (3,68) =5.6344, P =0.0017; 75–100 μm: F (3,61) =9.7476, P <0.0001, * P <0.05 versus control, Tukey–Kramer honestly significant difference post hoc ; n (neurons, subjects): Control (19,8), Nondep (24,9), DE (20,8), DE-RD (16,6). Full size image Parallel regulation of spine density in all cortical laminae One advantage of the DiOlistic method is that it allows tracking of dendritic spine density from neurons at all cortical depths. Therefore, we used DiOlistic labelling to test whether chronic monocular deprivation and subsequent recovery regulates the density of neuronal spines differently in neurons of different cortical lamina. Dendrites were sorted into three groups on the basis of the distance of the parent soma from the dura: 200–400 microns=superficial, 400–600 microns=middle and 650–850 microns=deep. Chronic monocular deprivation induced a significant, parallel decrease in spine density in all cortical laminae. No change was observed in the density of dendritic spines on neuron at any cortical depth following dark exposure alone. However, dark exposure followed by reverse deprivation significantly increased the density of dendritic spines at all cortical depths, including the middle lamina, which receives rich thalamic innervation (average normalized spine density±s.e.m. : superficial control=1.00±0.06 (7,4); chronic MD=0.55±0.11 (7,5); cMD DE=0.56±0.11(8,5); cMD DE-RD=0.81±0.19 (5,4); mid control=1.00±0.08 (5,4); chronic MD=0.59±0.10 (7,4); cMD DE=0.57±0.07 (6,4); cMD DE-RD=0.97±0.10 (5,3); deep control=1.00±0.06 (7,6); chronic MD=0.58±0.11 (10,5); cMD DE=0.45±0.14 (6,4); cMD DE-RD=0.83±0.11 (6,5); n =neurons, subjects; Fig. 4 ). Thus, the recovery from chronic monocular deprivation is accompanied by significant spinogenesis throughout the visual cortex, including the thalamo-recipient cortex. 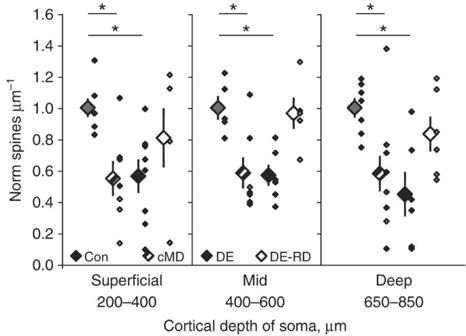Figure 4: Parallel regulation of dendritic spine density in all laminae of the deprived visual cortex. Chronic monocular deprivation (cMD) induces a significant decrease in dendritic spine density relative to binocular control (Con) in all cortical lamina. The reduction in dendritic spine density is unchanged following dark exposure (DE). Dark exposure and reverse deprivation (DE-RD) induce a significant increase in dendritic spine density in all cortical laminae (average normalized spine density±s.e.m.: one-way ANOVAs: superficial F(3,26)=3.7793,P=0.0243 (Con (7,4), cMD (7,5), DE (8,5), DE-RD (5,4)); mid F(3,22)=6.7756,P=0.0027 (Con (5,4), cMD (7,4), DE (6,4), DE-RD (5,3)); deep F(3,28)=4.5740,P=0.0110, (Con (7,6), cMD (10,5), DE (6,4), DE-RD (6,5)); *P<0.05 versus control, Tukey–Kramer honestly significant differencepost hoc;n(neurons, subjects)). Large symbols represent group average, small symbols represent data from individual neurons. Figure 4: Parallel regulation of dendritic spine density in all laminae of the deprived visual cortex. Chronic monocular deprivation (cMD) induces a significant decrease in dendritic spine density relative to binocular control (Con) in all cortical lamina. The reduction in dendritic spine density is unchanged following dark exposure (DE). Dark exposure and reverse deprivation (DE-RD) induce a significant increase in dendritic spine density in all cortical laminae (average normalized spine density±s.e.m. : one-way ANOVAs: superficial F (3,26) =3.7793, P =0.0243 (Con (7,4), cMD (7,5), DE (8,5), DE-RD (5,4)); mid F (3,22) =6.7756, P =0.0027 (Con (5,4), cMD (7,4), DE (6,4), DE-RD (5,3)); deep F (3,28) =4.5740, P =0.0110, (Con (7,6), cMD (10,5), DE (6,4), DE-RD (6,5)); * P <0.05 versus control, Tukey–Kramer honestly significant difference post hoc ; n (neurons, subjects)). Large symbols represent group average, small symbols represent data from individual neurons. Full size image Dark exposure reactivates plasticity at thalamocortical synapses Strengthening of thalamocortical synapses during the recovery from chronic monocular deprivation in adulthood would be unexpected. Although plasticity at thalamocortical synapses can be revealed by direct thalamic stimulation in vivo [37] , [38] , [39] , many reports have indicated that synaptic plasticity at thalamocortical synapses is constrained very early in postnatal development in many species [5] , [40] , [41] , [42] , [43] , [44] , [45] . Therefore, we used two complementary strategies to test the hypothesis that plasticity at thalamocortical synapses contributes to the recovery from chronic monocular deprivation in adulthood. First, we examined the regulation of ocular dominance of single units isolated from the thalamo-recipient zone of the primary visual cortex. We used the shape of the VEP waveform to guide electrode placement in layer IV [37] , [46] and simultaneously recorded VEPs (50 Hz low-pass filter) and neuronal spiking (300 Hz high-pass filter and a 3 kHz low-pass filter, Fig. 5a ). We observed the expected contralateral bias in the ocular dominance of single units acquired from the thalamo-recipient zone of control binocular adults [6] , [47] reflecting the complement of thalamocortical projections [48] . Chronic monocular deprivation shifted the ocular dominance of single units away from the deprived (contralateral) eye, and dark exposure followed by reverse deprivation in adulthood shifted ocular dominance back to control levels ( Fig. 5b–d ). The reversible change in the response properties of layer IV neuronal output was reflected in the contralateral bias index (CBI=[(N1–N5)+(N2–N4)+(Ntot/2Ntot)], where N(tot) is the total number of neurons, and N1–N5 represent the number of neurons in classes 1–5, as described in methods) and the average ocular dominance score (spike rate in response to stimulation of contra−ipsi eye/contra+ipsi eye±s.e.m. : control=0.25±0.08 (32,5); cMD=−0.05±0.09 (41,6); cMD DE-RD=0.32±0.08 (40,6); one-way ANOVA, F (2,112) =6.1897, P =0.0028, n =units, subjects). The cumulative distribution of ocular dominance scores revealed a significant rightward shift in the ocular preference of layer IV neurons away from the chronically deprived eye ( Fig. 5e , P =0.018, Kolmogorov–Smirnov (KS) test). Surprisingly, however, ∼ 34% of neurons retained ocular dominance scores >0.20 following chronic monocular deprivation, demonstrating the persistence of sensitivity to visual stimulation of the chronically deprived eye. Dark exposure and reverse deprivation induced a significant leftward shift in the ocular dominance scores, indicating increased sensitivity to stimulation of the previously deprived, contralateral eye ( Fig. 5f , P =0.007, KS test). Ocular dominance scores of chronically deprived subjects with dark exposure followed by reverse deprivation were indistinguishable from normal binocular controls ( Fig. 5g , P =0.322, KS test). 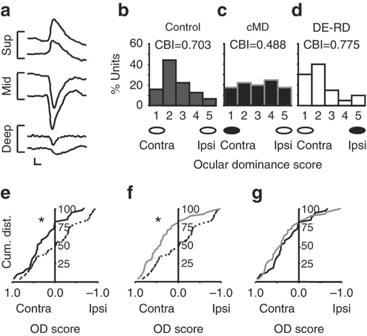Figure 5: Restoration of ocular dominance of single units isolated from thalamo-recipient cortex during the recovery from chronic monocular deprivation. (a) The shape of the VEP waveform changes as the recording electrode moves vertically through the cortex. VEPs are acquired with 50-Hz low-pass filter of evoked activity, and each waveform is an average of 100 presentations of 0.04 cycles/degree, 96% contrast horizontal gratings reversing at 1 Hz. Scale bars, 50 ms, 100 μV. A VEP with a large negative component confirms placement of the recording electrode in the thalamo-recipient cortex. (b) Unit activity from thalamo-recipient cortex was acquired with 300-Hz high-pass and a 3-kHz low-pass filter of evoked activity. (c) Chronic monocular deprivation (cMD) induces a shift in the ocular preference of single units away from the deprived eye (black oval) and towards the non-deprived eye (white oval). (d) Dark exposure and reverse deprivation (DE-RD) induce a shift back to normal contralateral preference. (b–d) Reversible change in contralateral bias index (CBI) also reflects the response to chronic monocular deprivation, and recovery following dark exposure and reverse deprivation. (e) Cumulative distribution (cum. dist.) of ocular dominance (OD) scores of single units obtained from thalamo-recipient cortex reveals a significant shift away from deprived (contralateral) eye following chronic monocular deprivation (dashed line) relative to binocular controls (black line; *P=0.018, KS test; control (32, 5), cMD (41,6);n(units, subjects)). (f) Significant reversal of the shift in OD scores towards the recovering (contralateral) eye following dark exposure and reverse deprivation (grey line) relative to chronic monocular deprivation (dashed line; *P=0.007, KS test; DE-RD (40,6)). (g) No difference in OD scores in binocular controls (black line) and subjects that received chronic monocular deprivation followed by dark exposure and reverse deprivation (grey line;P=0.322; KS test). Figure 5: Restoration of ocular dominance of single units isolated from thalamo-recipient cortex during the recovery from chronic monocular deprivation. ( a ) The shape of the VEP waveform changes as the recording electrode moves vertically through the cortex. VEPs are acquired with 50-Hz low-pass filter of evoked activity, and each waveform is an average of 100 presentations of 0.04 cycles/degree, 96% contrast horizontal gratings reversing at 1 Hz. Scale bars, 50 ms, 100 μV. A VEP with a large negative component confirms placement of the recording electrode in the thalamo-recipient cortex. ( b ) Unit activity from thalamo-recipient cortex was acquired with 300-Hz high-pass and a 3-kHz low-pass filter of evoked activity. ( c ) Chronic monocular deprivation (cMD) induces a shift in the ocular preference of single units away from the deprived eye (black oval) and towards the non-deprived eye (white oval). ( d ) Dark exposure and reverse deprivation (DE-RD) induce a shift back to normal contralateral preference. ( b – d ) Reversible change in contralateral bias index (CBI) also reflects the response to chronic monocular deprivation, and recovery following dark exposure and reverse deprivation. ( e ) Cumulative distribution (cum. dist.) of ocular dominance (OD) scores of single units obtained from thalamo-recipient cortex reveals a significant shift away from deprived (contralateral) eye following chronic monocular deprivation (dashed line) relative to binocular controls (black line; * P =0.018, KS test; control (32, 5), cMD (41,6); n (units, subjects)). ( f ) Significant reversal of the shift in OD scores towards the recovering (contralateral) eye following dark exposure and reverse deprivation (grey line) relative to chronic monocular deprivation (dashed line; * P =0.007, KS test; DE-RD (40,6)). ( g ) No difference in OD scores in binocular controls (black line) and subjects that received chronic monocular deprivation followed by dark exposure and reverse deprivation (grey line; P =0.322; KS test). Full size image The recovery of normal ocular dominance of neuronal output from the thalamo-recipient cortex suggests that enhancement of thalamocortical synaptic transmission may participate in the recovery from chronic monocular deprivation. However, changes in the spiking output of neurons in thalamo-recipient laminae may also reflect changes in the strength of cortico-cortical synaptic inputs. To distinguish between these possibilities, we used cortical silencing to pharmacologically isolate activity at thalamocortical synapses. A combination of the GABA A receptor agonist muscimol (4 mM, to hyperpolarize cortical neurons) and the GABA B receptor antagonist SCH50911 (6 mM, to block activation of presynaptic GABA B receptors by muscimol) delivered intracranially has recently been used to isolate the thalamocortical component of auditory and visually evoked potentials [49] , [50] . Musc+SCH (500 nl delivered intracranially, infused over ∼ 60 min) silenced cortical spiking ( Fig. 6a ) and induced a significant reduction in the VEP recorded from thalamo-recipient cortex (average-deprived eye VEP±s.e.m., predrug: 129.8±3.6 μV; post-drug: 39.8±11.8, n =4, P =0.004, paired t -test, Fig. 6b,c ). Visual stimulation of the chronically deprived eye continued to evoke a small thalamocortical VEP. Cortical spiking and VEP amplitude recovered following washout of Musc+SCH. Cortical silencing was also used to isolate the thalamocortical VEP in subjects receiving dark exposure followed by reverse deprivation, to promote the recovery from chronic monocular deprivation (average±s.e.m. : predrug VEP 323.3±48.5; postdrug VEP: 172.5±22.4, n =4, P =0.005, paired t -test). Dark exposure followed by reverse deprivation induced a significant increase in the amplitude of the thalamocortical VEP (average±s.e.m. cMD: 0.31±0.10; cMD DE-RD: 0.54±0.01; P =0.027, unpaired t -test, Fig. 6d ). The amplitude of the thalamocortical VEP recovered to the level observed in normal binocular controls (VEP amplitude postdrug/predrug, average±s.e.m. : 0.55±0.10, n =2, not shown). No nonspecific reduction in VEP amplitude or contralateral bias was observed in response to intracranial delivery of vehicle alone (postvehicle VEP amplitude normalized to prevehicle amplitude, average±s.e.m. : 0.93±0.05, n =2, paired t -test, P =0.13, not shown). Importantly, silencing cortical spiking did not reduce the VEP contralateral bias in adult rats, as previously reported in juvenile mice [50] (average VEP contralateral bias±s.e.m. cMD predrug: 0.38±0.070; postdrug: 0.38±0.12; cMD DE-RD predrug: 1.97±0.05; postdrug: 2.07±0.1; Fig. 6e ). 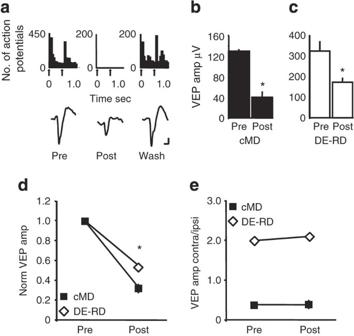Figure 6: Restoration of thalamocortical VEP amplitude during recovery from chronic monocular deprivation. (a) Representative VEP and unit activity (in 50 ms bins) evoked by visual stimulation before cortical silencing (pre; 0.04 cycle per degree. 96% contrast gratings at preferred orientation, reversing at 1 Hz, arrows). Intracortical infusion of muscimol+SCH50911 silences cortical spiking and reduces VEP amplitude (post). Cortical spiking and VEP amplitude recover following washout (∼10 h; wash). Scale bars, 50 ms, 50 μV. (b) Significant reduction in VEP amplitude following cortical silencing in subjects that received chronic monocular deprivation (cMD average deprived eye VEP±s.e.m.; *P=0.004, pairedt-test,n=4). (c) Significant reduction in VEP amplitude following cortical silencing in subjects that received chronic monocular deprivation followed by dark exposure and reverse deprivation (DE-RD average deprived eye VEP±s.e.m.; *P=0.005, pairedt-test;n=4). (d) Increase in the thalamocortical VEP amplitude following recovery from chronic monocular deprivation (normalized total VEP average±s.e.m.; *P=0.027, unpairedt-test). (e) Inhibition of cortical spiking does not modify the VEP contralateral bias in subjects that received chronic monocular deprivation, or chronic monocular deprivation followed by dark exposure and reverse deprivation. Figure 6: Restoration of thalamocortical VEP amplitude during recovery from chronic monocular deprivation. ( a ) Representative VEP and unit activity (in 50 ms bins) evoked by visual stimulation before cortical silencing (pre; 0.04 cycle per degree. 96% contrast gratings at preferred orientation, reversing at 1 Hz, arrows). Intracortical infusion of muscimol+SCH50911 silences cortical spiking and reduces VEP amplitude (post). Cortical spiking and VEP amplitude recover following washout ( ∼ 10 h; wash). Scale bars, 50 ms, 50 μV. ( b ) Significant reduction in VEP amplitude following cortical silencing in subjects that received chronic monocular deprivation (cMD average deprived eye VEP±s.e.m. ; * P =0.004, paired t -test, n =4). ( c ) Significant reduction in VEP amplitude following cortical silencing in subjects that received chronic monocular deprivation followed by dark exposure and reverse deprivation (DE-RD average deprived eye VEP±s.e.m. ; * P =0.005, paired t -test; n =4). ( d ) Increase in the thalamocortical VEP amplitude following recovery from chronic monocular deprivation (normalized total VEP average±s.e.m. ; * P =0.027, unpaired t -test). ( e ) Inhibition of cortical spiking does not modify the VEP contralateral bias in subjects that received chronic monocular deprivation, or chronic monocular deprivation followed by dark exposure and reverse deprivation. Full size image Chronic monocular deprivation induces severe amblyopia that is resistant to spontaneous reversal [51] . The obstacles to recovery include the developmental reduction in physiological and anatomical plasticity in the visual cortex, and the considerable degradation of feedforward excitation predicted to result from chronic monocular deprivation. Indeed, we show that chronic monocular deprivation induced a significant reduction in the density of basolateral dendritic spines of principal neurons throughout the deprived visual cortex. However, dark exposure followed by reverse deprivation in adulthood promotes the recovery from chronic monocular deprivation [27] . Indeed, dark exposure and reverse deprivation in adulthood stimulated an increase in dendritic spine density in neurons throughout the visual cortex. Importantly, dark exposure followed by reverse deprivation promotes the recovery of ocular dominance of neurons from the thalamo-recipient cortex, and the amplitude of the thalamocortical VEP. Thus, dark exposure in adulthood induces widespread anatomical and physiological plasticity at synapses throughout the visual cortex, including thalamocortical synapses, during the recovery from chronic monocular deprivation. The DiOlistic labelling technique allowed analysis of dendritic spine density throughout cortical lamina, and along the length of the basolateral dendrite. DiOlistic labelling revealed that the anatomical response to recovery from chronic monocular deprivation differed along the length of the basolateral dendrite. The recovery of dendritic spine density following dark exposure and reverse deprivation was greater in the proximal (0–75 μm from the soma) segment of the basolateral dendrite. This suggests that synapses in the proximal portion of the dendrite may have a lower threshold for experience-induced spinogenesis following dark exposure and reverse deprivation. Indeed, proximal synapses are more likely than distal to exhibit activity-dependent potentiation in response to the same stimulus parameters [52] . Enhancement of correlation-based plasticity and spinogenesis may be due to the higher concentration of voltage-gated sodium channels in proximal dendritic segments [53] . Chronic monocular deprivation in Long Evans rats induced a net reduction in dendritic spine density, suggesting that the depression and elimination of synapses serving the deprived eye dominates the response to prolonged monocular deprivation initiated in juveniles. Similarly, monocular deprivation (6–7 days) in kittens induces a decrease in the length of thalamocortical afferents serving the deprived eye [32] . However, the anatomical plasticity recruited by monocular deprivation in juvenile mice is biphasic. A rapid decrease in the density of spines on the apical dendrites of layer II/III pyramidal neurons is induced by brief monocular deprivation. Extending the duration of the monocular deprivation reveals a recovery of dendritic spine density. The strengthening of non-deprived eye responses [1] may promote the generation of new excitatory synapses [19] . Monocular deprivation in juvenile mice also induces a biphasic change in thalamocortical afferent number, such that an initial decrease in afferents serving the deprived eye is supplemented by a delayed increase in afferents serving the non-deprived eye [54] . Chronic monocular deprivation induced a decrease in dendritic spine density on principal neurons throughout the depth of the visual cortex. The parallel anatomical response in all cortical laminae is surprising given differences in the mechanisms of monocular-deprivation induced synaptic depression across layers of the visual cortex [4] , [47] , [55] . However, it is estimated that <10% of excitatory synapses onto principal neurons in layer IV originate from the thalamus in the cat [56] , and thalamic afferents are predicted to account for a similarly small complement of excitatory input onto thalamo-recipient neurons in the rodent. Therefore, the ∼ 50% decrease in dendritic spine density that we observed in response to chronic monocular deprivation may reflect depression and subsequent elimination of excitatory cortico-cortical synapses. We did not observe a decrease in the spine density on principal neurons in the visual cortex ipsilateral to the occlusion, suggesting that chronic deprivation of the non-dominant ipsilateral input did not trigger synaptic elimination. Contrary to our predictions, dark exposure alone did not induce a change in dendritic spine density or morphology in the visual cortex of chronically deprived adults. We also observed no compensatory changes in the morphology of residual spines that persisted following chronic monocular deprivation and dark exposure. Compensatory scaling of the density of dendritic spines may require a larger reduction in synaptic input [10] , [57] . Indeed, high levels of spontaneous synaptic input may suppress homeostatic scaling of spine density and morphology by dark exposure in chronically deprived adults. In contrast, dark exposure in adulthood may reactivate synaptic plasticity by enhancing the motility of residual spines. Indeed, dark-rearing mice until the peak of the critical period induces a persistent enhancement of the dynamics of dendritic spines on layer V pyramidal neurons [58] . Alternatively, regulation of dendritic spine density may require a competitive process, as observed following partial deprivation of neuronal input to multi-whisker septal neurons in the barrel cortex [10] and binocular neurons in the visual cortex [19] , [20] , [22] , [59] . Previous examinations of dendritic spine density by manipulation of visual experience in rodents have been limited to tracking anatomical changes in single cortical lamina [10] , [19] , [23] or dendritic compartments that receive substantial cortico-cortical excitatory input [20] . By tracking dendritic spines on pyramidal neurons throughout the depth of the visual cortex, we demonstrated a significant loss and recovery of dendritic spine density in all cortical laminae, including the thalamo-recipient zone. Although brief monocular deprivation in juveniles shifts the response properties of thalamo-recipient neurons [6] , [43] , [50] , receptive field plasticity at thalamocortical synapses is constrained very early in postnatal development [43] , [44] , [45] . Surprisingly, visual stimuli presented to the chronically deprived eye continued to evoke residual single unit activity in neurons from the thalamo-recipient cortex and a residual thalamocortical VEP, demonstrating the persistence of thalamocortical synaptic transmission following chronic monocular deprivation. The residual feedforward excitation likely provides the anatomical scaffold on which anatomical plasticity, once reactivated in the adult visual cortex by dark exposure, can promote the recovery from chronic monocular deprivation. In the absence of dark exposure, reverse deprivation does not promote the recovery of dendritic spine density or spatial acuity in rats [23] , [27] consistent with the absence of rapid anatomical and physiological plasticity in the adult rat visual cortex [60] . However, a significant increase in dendritic spine density was observed during the recovery from chronic monocular deprivation by dark exposure and reverse deprivation in adulthood. The new spines that emerge following dark exposure and reverse deprivation are likely to form functional synapses and contribute to the increase in the amplitude of the deprived eye VEP observed during the recovery from chronic monocular deprivation. The ocular dominance of neurons in thalamo-recipient laminae of the cortex and the amplitude of the thalamocortical VEP also recover when dark exposure is followed by reverse deprivation, indicating the strengthening of thalamocortical synapses. Thus, dark exposure in adulthood reactivates widespread anatomical and physiological plasticity in the visual cortex, including thalamocortical synapses, to promote the recovery from chronic monocular deprivation. Subjects Long Evans rats (equal numbers of males and females) received chronic monocular deprivation via lid suture, from eye opening (approximately postnatal day 14) to adulthood (average±s.e.m. age at experiment postnatal day 148±11.65). In some cases, chronic monocular deprivation was followed by 10 days of dark exposure±7 days of reverse deprivation (opening chronically deprived eye and suturing non-deprived eye). Control subjects (equal numbers of males and females) were raised in a normal visual environment (12 h light/12 h dark per day), and all subjects had food and water available ad libitum . All procedures conformed to the guidelines of the US Department of Health and Human Services and the University of Maryland Institutional Animal Care and Use Committee. Anatomy A modification of the DiOlistic staining method of Gan et al . [35] was used. Briefly, transcardial perfusion (100 ml, 2% paraformaldehyde in 0.1 M phosphate buffer, pH 7.3) was followed by postfixation of the brain (1 h in 2% paraformaldehyde at room temperature (RT)). Coronal sections of visual cortex (200 μm thickness) were prepared in ice-cold phosphate-buffered saline (PBS, pH 7.3) on a vibratome. The lipophilic dye, DiI (1,1′-dioctadecyl-3,3,3′,3′-tetramethylindocarbocyanine perchlorate), was coated onto tungsten particles (1.3 μm) and delivered into slices with a Helios gene gun (Bio-Rad; 60–80 psi helium pressure). Cortical slices were incubated in PBS (2.5 h at RT) to allow the dye to diffuse, followed by a second postfix (4% paraformaldehyde for 30 min at RT). Slices were mounted in ProLong gold antifade reagent (Invitrogen). Neuronal selection within the binocular region of the visual cortex was based on characteristic pyramidal soma, distinct basolateral and apical dendrites at low magnification (×10), as dendritic spines are not detectable at this magnification. Only one basolateral dendrite was scored per neuron. Neurons were sorted into categories (superficial, mid and deep) based on depth of the parent cell body from the dura and other identifying landmarks. Confocal images were acquired using a Zeiss 710 confocal microscope. A typical z-stack consisted of ∼ 30 optical image planes each of 436×436 pixels. We used a 63×/1.4 Oil DIC Plan Apo objective with ×3 zoom with 0.42 μm z-steps. Images were acquired with a 63×/1.4 Oil DIC Plan Apo objective with ×3 zoom with 0.42 μm z-steps. Maximum intensity projections were exported and photomontages were constructed in Photoshop (Adobe), and images were calibrated and quantified using an image processing toolkit (Reindeer graphics). All protrusions with a neck and head were manually marked and quantified using 'Count' function. Lines tracing the head diameters and neck length (as demonstrated in Fig. 2 ) were drawn on each spine and lengths calculated with 'Measure all features' function. An observer who was blind to the experimental condition analysed a subset of the morphological data. Physiology Visually evoked potentials were recorded from the thalamo-recipient laminae ( ∼ 500 microns from the dural surface) of the binocular visual cortex (7 mm posterior of bregma, 4 mm lateral of midline) with tungsten microelectrodes (1 MΩ), following urethane anaesthesia (1.4 mg kg −1 , intraperitoneal). Visual stimuli were 1 Hz full-screen square-wave gratings with a spatial frequency of 0.02–0.04 cycles per degree, 96% maximal contrast and 25 cd m −2 luminance. The amplitude of the primary negative (thalamo recipient) component of the evoked potential was quantified to assess the cortical response to visual stimulation. VEP waveforms were averaged from 100 visual stimuli presentations. Subdural electrode placement allowed for the simultaneous collection of thalamo-recipient VEPs (50 Hz low-pass filter) and neuronal spiking (300 Hz high pass and a 3 kHz low pass) in response to visual stimulation. Multiunit activity was sorted into single units on the basis of waveform shape and principal component analysis using OpenEx software (TDT). Ocular dominance scores were calculated on the basis of individual eye peak activity responses in poststimulus time histograms (contra eye−ipsi eye)/(contra eye+ipsi eye) and were binned in a modified version of the classic scale introduced by Hubel and Wiesel: 1=1.00–0.60, 2=0.59–0.20, 3=0.19 to −0.19, 4=−0.20 to −0.59, 5=−0.60 to −1.00, where 1 represents units primarily driven by the contralateral eye and 5 represents units primarily driven by the ipsilateral eye. Contralateral bias index was calculated by using the formula [(N1–N5)+(N2–N4)+(Ntot/2Ntot)], where N(tot) is the total number of cells and N1–5 is the number of neurons in bins 1–5, respectively. The thalamocortical location of the electrode was confirmed anatomically by a post hoc reconstruction of the electrode track. Before transcardial perfusion (4% paraformaldehyde), the electrode was cemented to the skull with dental acrylic to maintain electrode placement during fixation. Following overnight postfix (4% paraformaldehyde), coronal sections (50 microns) were collected on a vibratome in PBS. A cresyl violet nissl stain was used to reveal the laminar organization of the visual cortex, and the placement of the recording electrode in layer IV. Brightfield images ( Fig. 1b ) were collected on a Zeiss 710 confocal microscope in transmitted light mode using a ×10 air objective. A photomontage was constructed in Photoshop to reveal the laminar location of the electrode track. Only contrast or brightness was adjusted as needed for the photomontage. Pharmacology The thalamocortical component of the VEP was isolated using a combination of the GABA A receptor agonist muscimol (4 mM, to silence cortical spiking) and the GABA B receptor antagonist SCH50911 (6 mM, to prevent activation of presynaptic GABA B receptors) as described [49] , [50] . A small craniotomy was made ∼ 500 microns posterior to the recording craniotomy (7 mm posterior of bregma, 4 mm lateral of midline). The drug or ACSF (artificial cerebrospinal fluid) was delivered intracranially ( ∼ 500 nl) through a guide cannula (26 gauge, Plastics One; attached to surrounding skull with dental acrylic) allowed to infuse for ∼ 60 min. Statistics One-way ANOVA was used to determine statistical significance between three or more independent experimental groups ( P <0.05). A subsequent Tukey–Kramer honestly significant difference post hoc analysis was used to make pairwise comparisons (JMP). A KS test was used to determine statistical significance in the distribution of two independent data sets ( P <0.05). A paired or unpaired t -test was used to probe the statistical significance for two experimental groups ( P <0.05). How to cite this article: Montey, K. L. & Quinlan, E.M. Recovery from chronic monocular deprivation following reactivation of thalamocortical plasticity by dark exposure. Nat. Commun. 2:317 doi: 10.1038/ncomms1312 (2011).